Tumour-associated mutant p53 drives the Warburg effect Tumour cells primarily utilize aerobic glycolysis for energy production, a phenomenon known as the Warburg effect. Its mechanism is not well understood. The tumour suppressor gene p53 is frequently mutated in tumours. Many tumour-associated mutant p53 (mutp53) proteins not only lose tumour suppressive function but also gain new oncogenic functions that are independent of wild-type p53, defined as mutp53 gain of function (GOF). Here we show that tumour-associated mutp53 stimulates the Warburg effect in cultured cells and mutp53 knockin mice as a new mutp53 GOF. Mutp53 stimulates the Warburg effect through promoting GLUT1 translocation to the plasma membrane, which is mediated by activated RhoA and its downstream effector ROCK. Inhibition of RhoA/ROCK/GLUT1 signalling largely abolishes mutp53 GOF in stimulating the Warburg effect. Furthermore, inhibition of glycolysis in tumour cells greatly compromises mutp53 GOF in promoting tumorigenesis. Thus, our results reveal a new mutp53 GOF and a mechanism for controlling the Warburg effect. Tumour suppressor p53 has a central role in tumour prevention [1] , [2] , [3] . p53 is the most frequently mutated gene in human tumours. Majority of p53 mutations, including several ‘mutational hotspots’ in tumours (for example, R175H, R248Q and R273H), are missense mutations, which usually result in the expression of full-length mutant p53 (mutp53) proteins in tumour cells. Recent studies have demonstrated that many tumour-associated mutp53 proteins, particularly these several ‘tumour hotspot mutants’, not only lose tumour suppressive functions of wild-type p53 (wtp53) but also gain new oncogenic functions that are independent of wtp53, including promoting cell proliferation, anti-apoptosis and metastasis, which are defined as mutp53 gain of function (GOF) [4] , [5] , [6] , [7] . The mutp53 GOF is clearly demonstrated by mutp53 knockin mouse models; mice that express R172H or R270H mutp53 (equivalent to human R175H and R273H, respectively) develop an altered spectrum of tumours and more metastatic tumours compared with p53−/− mice [8] , [9] . The mechanism of mutp53 GOF in tumorigenesis is not well understood. Recent studies have shown that metabolic changes are a hallmark of tumour cells and a key contributor to tumour development [10] , [11] , [12] , [13] . The Warburg effect (or aerobic glycolysis) is the best-characterized metabolic change in tumour cells. Most tumour cells primarily utilize glycolysis for their energy needs even under normal oxygen concentrations, a phenomenon termed ‘the Warburg effect’ [14] . The Warburg effect is characterized by a much higher rate of glucose uptake and higher lactate production in tumour cells compared with normal cells [10] , [12] , [13] , [14] . The Warburg effect provides a rational for positron emission tomography imaging developed for tumour detection, as tumours take up more of the glucose analogue 18 fluorodeoxyglucose than normal tissues. Emerging evidence has indicated that the Warburg effect contributes greatly to tumorigenesis and could be targeted for tumour therapy [12] , [15] , [16] . However, the mechanism for the Warburg effect is not well understood. As a transcription factor, wtp53 mainly exerts its function in tumour suppression through transcriptional regulation of its target genes to initiate various cellular responses, including cell cycle arrest and apoptosis [1] , [2] , [3] . Recent studies have shown that regulating energy metabolism is a critical function of wtp53 in tumour suppression [12] , [13] , [17] , [18] . Wtp53 represses glycolysis and the Warburg effect through transcriptional regulation of genes involved in energy metabolism, including SCO2 , TIGAR , GLS2 and Parkin [19] , [20] , [21] , [22] . Loss of wtp53 leads to the Warburg effect in cultured cells and mice. It remains unknown whether mutp53 can stimulate the Warburg effect as a novel GOF. In this study, we find that tumour-associated mutp53 stimulates the Warburg effect both in cultured cells and mutp53 knockin mice. This effect is achieved mainly through promoting the translocation of GLUT1 (glucose transporter 1) to the plasma membrane (PM), which is mediated by an activated RhoA/ROCK (Rho-associated protein kinase) signalling. Inhibition of glycolysis and the Warburg effect in tumour cells greatly attenuates mutp53 GOF in tumorigenesis. Our results demonstrate a new mutp53 GOF and also reveal a new mechanism for the Warburg effect in cancer cells. Mutp53 stimulates the Warburg Effect in vitro and in vivo The Warburg effect is characterized by greatly increased glucose uptake and lactate production in tumour cells [12] , [14] . To investigate the effect of mutp53 on the Warburg effect, p53-null human lung carcinoma H1299 cells were stably transduced with retroviral vectors expressing ‘tumour hotspot mutants’ R175H, R248Q and R273H mutp53, and the levels of glucose uptake, glycolytic rate and lactate production in cells were measured. Expression of R175H, R248Q and R273H mutp53 in H1299 cells greatly stimulated the Warburg effect; much higher levels of glucose uptake, glycolytic rate and lactate production were observed in cells with mutp53 expression compared with that in control cells ( Fig. 1a ). A similar effect was observed for endogenous mutp53; in human breast SK-BR3 and MDA-MB468 cells, which express R175H and R273H mutp53, respectively, knockdown of endogenous mutp53 by short hairpin RNA (shRNA) vectors greatly reduced glucose uptake, glycolytic rate and lactate production ( Fig. 1b ). This stimulating effect of mutp53 on the Warburg effect was also observed in mouse embryonic fibroblasts (MEFs) from p53 R172H/R172H knockin mice (equivalent to human R175H ). Compared with p53−/− MEFs, p53 R172H/R172H MEFs showed clearly enhanced glucose uptake, glycolytic rate and lactate production ( Fig. 1c ). Furthermore, the enhanced glucose uptake was observed in different tissues in p53 R172H/R172H mice compared with p53−/− mice, including the liver, lung and small intestine ( Fig. 1d ). It is well-established that the serum lactate level indicates glycolytic status in mice [23] , [24] . p53 R172H/R172H mice showed much higher levels of serum lactate than p53−/− mice ( Fig. 1e ), indicating a higher glycolytic rate in p53 R172H/R172H mice. 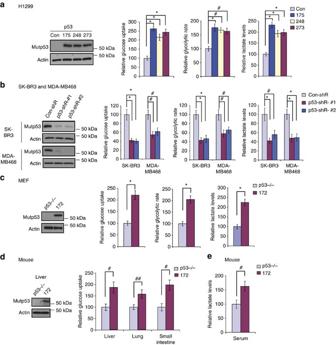Figure 1: Mutp53 stimulates the Warburg effect bothin vitroandin vivo. (a) Ectopic expression of R175H, R248Q and R273H mutp53 in p53-null H1299 cells enhanced glucose uptake, glycolytic rate and lactate production. Con: Control. Left panels ina–d: mutp53 expression in cells detected by western blotting assays. (b) Knockdown of endogenous mutp53 by two different shRNA vectors in SK-BR3 cells expressing R175H mutp53 and MDA-MB468 cells expressing R273H mutp53 reduced glucose uptake, glycolytic rate and lactate production. Con-shR, control shRNA; p53-shR, p53 shRNA. (c) Enhanced glucose uptake, glycolytic rate and lactate production inp53R172H/R172HMEFs compared withp53−/−MEFs. 172:p53R172H/R172H. (d) Increased glucose uptake in different tissues inp53R172H/R172Hmice compared withp53−/−mice. (e) Increased serum lactate levels inp53R172H/R172Hmice compared withp53−/−mice. Data are presented as mean±s.d. (n=5 fora–c,n=6 ford,e).##P<0.05;#P<0.01; *P<0.005; two-tailed Student’st-test. Figure 1: Mutp53 stimulates the Warburg effect both in vitro and in vivo . ( a ) Ectopic expression of R175H, R248Q and R273H mutp53 in p53-null H1299 cells enhanced glucose uptake, glycolytic rate and lactate production. Con: Control. Left panels in a – d : mutp53 expression in cells detected by western blotting assays. ( b ) Knockdown of endogenous mutp53 by two different shRNA vectors in SK-BR3 cells expressing R175H mutp53 and MDA-MB468 cells expressing R273H mutp53 reduced glucose uptake, glycolytic rate and lactate production. Con-shR, control shRNA; p53-shR, p53 shRNA. ( c ) Enhanced glucose uptake, glycolytic rate and lactate production in p53 R172H/R172H MEFs compared with p53−/− MEFs. 172: p53 R172H/R172H . ( d ) Increased glucose uptake in different tissues in p53 R172H/R172H mice compared with p53−/− mice. ( e ) Increased serum lactate levels in p53 R172H/R172H mice compared with p53−/− mice. Data are presented as mean±s.d. ( n =5 for a – c , n =6 for d , e ). ## P <0.05; # P <0.01; * P <0.005; two-tailed Student’s t -test. Full size image Recently, wtp53 was reported to repress the Warburg effect [19] , [20] , [21] . To further confirm that this stimulating effect of mutp53 on the Warburg effect is a novel mutp53 GOF and is independent of the function of wtp53, we examined whether wtp53 exhibits an inhibitory effect on the Warburg effect as reported using our systems. As shown in Fig. 2a , p53+/+ MEFs displayed much lower levels of glucose uptake, glycolytic rate and lactate production than p53−/− MEFs. Consistently, compared with p53−/− mice, p53+/+ mice displayed a much lower level of glucose uptake in different tissues ( Fig. 2b ) and a clear lower level of serum lactate ( Fig. 2c ). Furthermore, knockdown of endogenous wtp53 by shRNA vectors in human breast MCF7, lung H460 and A549 cells clearly promoted the glucose uptake, glycolytic rate and lactate production compared with control cells transduced with control shRNA vectors ( Fig. 2d ). These results clearly show that wtp53 can repress the Warburg effect in vitro and in vivo , which is consistent with previous reports [19] , [20] , [21] . Thus, our results clearly demonstrate that stimulating the Warburg effect is a novel mutp53 GOF, which is independent of wtp53’s function. 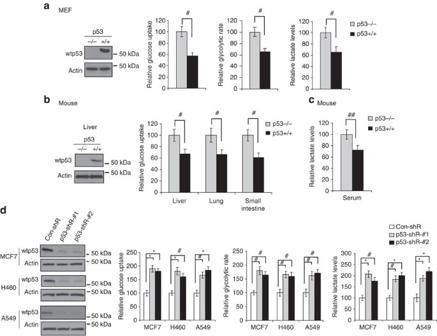Figure 2: Wild-type p53 inhibits the Warburg effect bothin vitroandin vivo. (a) Lower levels of glucose uptake, glycolytic rate and lactate production inp53+/+MEF cells compared withp53−/−MEF cells. wtp53: wild-type p53. (b) Lower levels of glucose uptake in different tissues inp53+/+mice compared withp53−/−mice. (c) Lower levels of serum lactate inp53+/+mice compared withp53−/−mice. (d) Knockdown of the endogenous wtp53 by two different shRNA vectors in human breast MCF7, human lung H460 and A549 cells, which all express wtp53, enhanced glucose uptake, glycolytic rate and lactate production in cells. Con-shR, control shRNA; p53-shR, p53 shRNA. Left panels ina,bandd: wtp53 expression in cells detected by western blotting assays. Data are presented as mean±s.d. (n=4 fora,d,n=6 forb,c).##P<0.05;#P<0.01; *P<0.005; two-tailed Student’st-test. Figure 2: Wild-type p53 inhibits the Warburg effect both in vitro and in vivo . ( a ) Lower levels of glucose uptake, glycolytic rate and lactate production in p53+/+ MEF cells compared with p53−/− MEF cells. wtp53: wild-type p53. ( b ) Lower levels of glucose uptake in different tissues in p53+/+ mice compared with p53−/− mice. ( c ) Lower levels of serum lactate in p53+/+ mice compared with p53−/− mice. ( d ) Knockdown of the endogenous wtp53 by two different shRNA vectors in human breast MCF7, human lung H460 and A549 cells, which all express wtp53, enhanced glucose uptake, glycolytic rate and lactate production in cells. Con-shR, control shRNA; p53-shR, p53 shRNA. Left panels in a , b and d : wtp53 expression in cells detected by western blotting assays. Data are presented as mean±s.d. ( n =4 for a , d , n =6 for b , c ). ## P <0.05; # P <0.01; * P <0.005; two-tailed Student’s t -test. Full size image Mutp53 promotes GLUT1 translocation Transport of glucose across the PM of cells is the first rate-limiting step for glucose metabolism, which is mediated by glucose transporters (GLUTs), including GLUT1–4. GLUT4 is the main glucose transporter expressed in insulin-responsive fat and muscle tissues. Insulin dramatically stimulates the translocation of GLUT4 to the PM to promote the glucose uptake in fat and muscle. GLUT1–3 are responsible for the basal glucose uptake in cells and tissues [25] . Among them, GLUT1 is widely expressed in almost all types of cells and tissues, and is responsible for their basal glucose uptake, whereas GLUT2 and 3 are responsible for the basal glucose uptake in some specific tissues [25] . Whereas the dysregulation of GLUT4 signalling is an important cause for type 2 diabetes, dysregulation of GLUT1–3 signalling, especially GLUT1, contributes to tumorigenesis. For example, GLUT1 is frequently overexpressed in tumours, which contributes to the Warburg effect [26] , [27] . Indeed, ectopic expression of GLUT1 by expression vectors in H1299 and p53−/− MEF cells greatly enhanced glucose uptake, glycolytic rate and lactate production in cells ( Supplementary Fig. S1a–d ). It has been well-established that increased translocation of GLUT1 from the intracellular pool to the PM promotes glucose transport [25] , [28] . Interestingly, mutp53 promoted GLUT1 translocation to the PM in cells. Ectopic expression of mutp53 greatly increased GLUT1 levels on the PM but did not change the total GLUT1 levels in H1299 cells as measured by western blotting assays using isolated PM fractions ( Fig. 3a ). To confirm this result, cells were transduced with pLPCX-Myc-GLUT1 vectors expressing GLUT1 with Myc tag in its first exofacial loop, and the levels of Myc-GLUT1 on the cell surface or in the whole cell were measured by immunofluoroscence (IF) staining with an anti-Myc antibody followed by flow cytometry analysis. Mutp53 clearly increased the levels of Myc-GLUT1 protein on the PM but did not affect the total Myc-GLUT1 levels in H1299 cells ( Fig. 3b ). Similar results were observed by IF staining of cells transduced with pLPCX-Myc-GLUT1 vectors; mutp53 expression in H1299 clearly promoted the translocation of Myc-GLUT1 protein from cytoplasm to the cell surface ( Fig. 3c ). Furthermore, knockdown of endogenous mutp53 in SK-BR3 and MDA-MB468 cells clearly reduced the levels of endogenous GLUT1 on the PM but not the total GLUT1 levels in the cells as analysed by western blotting assays ( Fig. 3d ), and reduced the levels of exogenous Myc-GLUT1 on the PM but not the total Myc-GLUT1 levels in the cells as analysed by IF assays in a flow cytometry ( Fig. 3e ). IF staining showed that mutp53 knockdown in both cell lines clearly decreased Myc-GLUT1 distribution on the cell surface and increased its distribution in the cytoplasm ( Fig. 3f ). 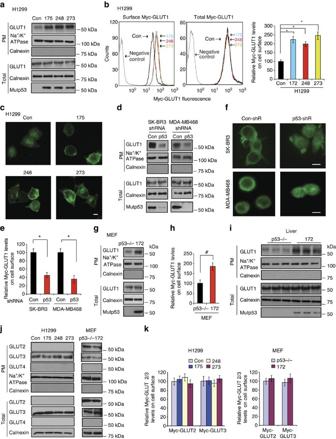Figure 3: Mutp53 stimulates GLUT1 translocation to the PM bothin vitroand invivo. (a) Ectopic expression of R175H, R248Q and R273H mutp53 in H1299 cells promoted GLUT1 translocation to the PM detected by western blotting assays. The PM protein Na+/K+ATPase acts as a loading control and Calnexin acts as a negative control for the PM fraction. Total, whole-cell lysates. (b) Mutp53 promoted Myc-GLUT1 translocation to the PM in H1299 cells analysed in a flow cytometry. Left and middle panels: represented images of fluorescence staining of Myc-GLUT1 on cell surface (left) and in the whole cell (middle). Right panel: relative Myc-GLUT1 levels on cell surface after normalization with the total Myc-GLUT1 levels in cells. Cells were transduced with pLPCX-Myc-GLUT1 vectors or pLPCX vectors (as negative controls) 48 h before assays. (c) IF staining of Myc-GLUT1 in H1299 control cells and cells with ectopic expression of R175H, R248Q or R273H mutp53. Scale bar, 10 μm. (d,e) Knockdown of endogenous mutp53 by shRNA in SK-BR3 and MDA-MB468 cells reduced the translocation of endogenous GLUT1 as measured by western blotting assays (d) and the translocation of Myc-GLUT1 to the PM measured by a flow cytometry (e). (f) IF staining of the Myc-GLUT1 in SK-BR3 and MDA-MB468 cells with mutp53 knockdown and control cells. Scale bar, 10 μm. Ind–f, two shRNA vectors against p53 were used and similar results were observed. (g,h) R172H mutp53 promoted the translocation of endogenous GLUT1 to the PM measured by western blotting assays (g) and Myc-GLUT1 to the PM analysed by a flow cytometry (h) inp53R172H/R172HMEF cells. (i) Higher endogenous GLUT1 levels on the PM in the liver tissues ofp53R172H/R172Hmice compared withp53−/−mice detected by western blotting assays. Six mice per group were analysed and three mice per group were presented. (j) Mutp53 did not promote the translocation or the expression of endogenous GLUT2 or GLUT3 in H1299 or MEF cells. (k) Mutp53 did not promote the PM translocation of Myc-GLUT2 or Myc-GLUT3 in H1299 and MEF cells analysed by a flow cytometry. Cells were transduced with pLPCX-Myc-GLUT2 or GLUT3 vectors at 48 h before assays. Data are presented as mean±s.d. (n=4). *P<0.005;#P<0.01; two-tailed Student’st-test. Figure 3: Mutp53 stimulates GLUT1 translocation to the PM both in vitro and in vivo . ( a ) Ectopic expression of R175H, R248Q and R273H mutp53 in H1299 cells promoted GLUT1 translocation to the PM detected by western blotting assays. The PM protein Na + /K + ATPase acts as a loading control and Calnexin acts as a negative control for the PM fraction. Total, whole-cell lysates. ( b ) Mutp53 promoted Myc-GLUT1 translocation to the PM in H1299 cells analysed in a flow cytometry. Left and middle panels: represented images of fluorescence staining of Myc-GLUT1 on cell surface (left) and in the whole cell (middle). Right panel: relative Myc-GLUT1 levels on cell surface after normalization with the total Myc-GLUT1 levels in cells. Cells were transduced with pLPCX-Myc-GLUT1 vectors or pLPCX vectors (as negative controls) 48 h before assays. ( c ) IF staining of Myc-GLUT1 in H1299 control cells and cells with ectopic expression of R175H, R248Q or R273H mutp53. Scale bar, 10 μm. ( d , e ) Knockdown of endogenous mutp53 by shRNA in SK-BR3 and MDA-MB468 cells reduced the translocation of endogenous GLUT1 as measured by western blotting assays ( d ) and the translocation of Myc-GLUT1 to the PM measured by a flow cytometry ( e ). ( f ) IF staining of the Myc-GLUT1 in SK-BR3 and MDA-MB468 cells with mutp53 knockdown and control cells. Scale bar, 10 μm. In d – f , two shRNA vectors against p53 were used and similar results were observed. ( g , h ) R172H mutp53 promoted the translocation of endogenous GLUT1 to the PM measured by western blotting assays ( g ) and Myc-GLUT1 to the PM analysed by a flow cytometry ( h ) in p53 R172H/R172H MEF cells. ( i ) Higher endogenous GLUT1 levels on the PM in the liver tissues of p53 R172H/R172H mice compared with p53−/− mice detected by western blotting assays. Six mice per group were analysed and three mice per group were presented. ( j ) Mutp53 did not promote the translocation or the expression of endogenous GLUT2 or GLUT3 in H1299 or MEF cells. ( k ) Mutp53 did not promote the PM translocation of Myc-GLUT2 or Myc-GLUT3 in H1299 and MEF cells analysed by a flow cytometry. Cells were transduced with pLPCX-Myc-GLUT2 or GLUT3 vectors at 48 h before assays. Data are presented as mean±s.d. ( n =4). * P <0.005; # P <0.01; two-tailed Student’s t -test. Full size image Consistent results were observed in p53 R172H/R172H MEF cells; R172H mutp53 clearly promoted the translocation of both endogenous GLUT1 and Myc-GLUT1 in MEF cells ( Fig. 3g,h ). Similar results were observed in p53 R172H/R172H mice; compared with p53−/− mice, mutp53 clearly increased GLUT1 levels on the PM but not the total GLUT1 levels in different tissues from p53 R172H/R172H mice, including the liver ( Fig. 3i ), lung and small intestine tissues ( Supplementary Fig. S2 ). Interestingly, mutp53 did not affect the translocation of GLUT2 or GLUT3, the other two glucose transporters that regulate the basal glucose uptake in certain types of tissues and cells. Expression of R175H, R248Q or R273H mutp53 in H1299 cells or R172H mutp53 in p53 R172H/R172H MEFs did not affect the levels of endogenous GLUT2/3 or Myc-GLUT2/3 on the PM or in the whole cell compared with control H1299 cells and p53−/− MEFs cells, respectively ( Fig. 3j,k ). The expression of GLUT4 and its translocation to the PM were also examined in H1299 and p53 R172H/R172H MEF cells. The levels of GLUT4 were too low to be detected in these two cell lines ( Fig. 3j ), indicating that GLUT4 is not a major contributor to the role of mutp53 in stimulating the Warburg effect in these cells. To test whether the enhanced GLUT1 translocation mediates the stimulating effect of mutp53 on the Warburg effect, endogenous GLUT1 was knocked down by shRNA or small interfering RNA (siRNA) oligos in cells. Whereas GLUT1 overexpression promotes the Warburg effect ( Supplementary Fig. S1 ), GLUT1 knockdown clearly reduced the glucose uptake, glycolytic rate and lactate production in H1299 and MEF cells ( Fig. 4a,b ). Notably, GLUT1 knockdown largely abolished the stimulating effect of mutp53 on the Warburg effect in H1299 cells and in p53 R172H/R172H MEF cells ( Fig. 4a,b ). In SK-BR3 and MDA-MB468 cells, GLUT1 knockdown clearly reduced the Warburg effect, similar to the effect of mutp53 knockdown ( Fig. 4c ). However, simultaneous knockdown of mutp53 and GLUT1 in these two cell lines did not produce additive inhibitory effect on the Warburg effect ( Fig. 4c ), further suggesting that GLUT1 mediates the stimulating effect of mutp53 on the Warburg effect in cells. 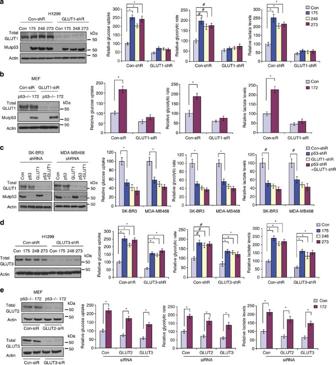Figure 4: GLUT1 mediates the stimulating effect of mutp53 on the Warburg effect in cells. (a) GLUT1 knockdown by shRNA vectors largely abolished the stimulating effects of R175H, R248Q and R273H mutp53 on the Warburg effect in H1299 cells. Con-shR, control shRNA; GLUT1-shR, GLUT1 shRNA. (b) GLUT1 knockdown by siRNA abolished the stimulating effect of R172H mutp53 on the Warburg effect in p53R172H/R172HMEFs. (c) GLUT1 knockdown by shRNA abolished the stimulating effect of R175H and R273H mutp53 on the Warburg effect in SK-BR3 and MDA-MB468 cells, respectively. (d) GLUT3 knockdown by shRNA did not clearly affect the stimulating effects of mutp53 on the Warburg effect in H1299 cells. Only GLUT3 was knocked down in H1299 cells, as GLUT2 expression was undetectable in H1299 (Fig. 3j). (e) Knockdown of GLUT2 or GLUT3 by siRNA did not clearly affect the stimulating effect of R172H mutp53 on the Warburg effect inp53R172H/R172HMEFs. Left panels ina–e: knockdown of GLUT1, GLUT2, or GLUT3 in cells analysed by western blotting assays. Two different shRNA vectors or siRNA oligos against GLUT1, 2 and 3, respectively, were used ina–e, and similar results were observed. Data are presented as mean±s.d. (n=3).#P<0.01; *P<0.005; two-tailed Student’st-test. Figure 4: GLUT1 mediates the stimulating effect of mutp53 on the Warburg effect in cells. ( a ) GLUT1 knockdown by shRNA vectors largely abolished the stimulating effects of R175H, R248Q and R273H mutp53 on the Warburg effect in H1299 cells. Con-shR, control shRNA; GLUT1-shR, GLUT1 shRNA. ( b ) GLUT1 knockdown by siRNA abolished the stimulating effect of R172H mutp53 on the Warburg effect in p53 R172H/R172H MEFs. ( c ) GLUT1 knockdown by shRNA abolished the stimulating effect of R175H and R273H mutp53 on the Warburg effect in SK-BR3 and MDA-MB468 cells, respectively. ( d ) GLUT3 knockdown by shRNA did not clearly affect the stimulating effects of mutp53 on the Warburg effect in H1299 cells. Only GLUT3 was knocked down in H1299 cells, as GLUT2 expression was undetectable in H1299 ( Fig. 3j ). ( e ) Knockdown of GLUT2 or GLUT3 by siRNA did not clearly affect the stimulating effect of R172H mutp53 on the Warburg effect in p53 R172H/R172H MEFs. Left panels in a – e : knockdown of GLUT1, GLUT2, or GLUT3 in cells analysed by western blotting assays. Two different shRNA vectors or siRNA oligos against GLUT1, 2 and 3, respectively, were used in a – e , and similar results were observed. Data are presented as mean±s.d. ( n =3). # P <0.01; * P <0.005; two-tailed Student’s t -test. Full size image Similar to the effect of GLUT1 knockdown on the Warburg effect, knockdown of endogenous GLUT3 by shRNA vectors or siRNA oligos in H1299 and MEFs greatly reduced glucose uptake, glycolytic rate and lactate production ( Fig. 4d,e ). However, GLUT3 knockdown did not clearly affect the promoting effect of mutp53 on the Warburg effect, which was still clearly observed in both cell lines with lower glycolytic rates caused by GLUT3 knockdown ( Fig. 4d,e ). Similarly, knockdown of GLUT2 clearly reduced the Warburg effect in both p53 −/− and p53 R172H/R172H MEFs, but did not clearly affect the promoting effect of mutp53 on the Warburg effect ( Fig. 4e ). These results strongly suggest that the promoting effect of mutp53 on the Warburg effect is mediated by GLUT1. Taken together, these results indicate that mutp53 can specifically promote GLUT1 translocation to the PM, which is an important mechanism for mutp53 to stimulate the Warburg effect in tumour cells. Mutp53 stimulates the Warburg effect through RhoA activation Small GTPase proteins, such as Rab and Rho families, were reported to be involved in the regulation of insulin-stimulated GLUT4 translocation to the PM and insulin-stimulated glucose uptake in fat and muscle, two insulin-responsive tissues [25] , [29] . RhoA is a small GTPase that belongs to the Rho family. RhoA is frequently overexpressed or activated in tumours and contributes to tumorigenesis by promoting proliferation and metastasis of tumour cells [30] , [31] . RhoA is also involved in stimulating GLUT4 translocation to the PM in response to insulin stimulation in fat and muscle cells [32] , [33] . Interestingly, mutp53 was recently reported to activate RhoA through its upregulation of the expression of positive regulators for RhoA, including RhoGDI and Rho GEF-H1 (refs 34 , 35 , 36 , 37 ). These findings raised a possibility that mutp53 may promote GLUT1 translocation and stimulate the Warburg effect through its activation of RhoA in tumour cells. However, the translocation regulation of GLUT1 and GLUT4 in cells is quite different, which is highly cell-type specific [25] , [32] . For example, the translocation of GLUT4 is dramatically stimulated by insulin, whereas GLUT1 translocation is not markedly regulated by insulin [25] , [32] . Currently, it is unclear whether RhoA can regulate GLUT1 translocation to affect the basal glucose uptake, and whether RhoA activation can promote the Warburg effect in cancer cells. We first tested whether mutp53 activates RhoA in the cells we used for this study. RhoA cycles between inactive GDP-bound and active GTP-bound states in cells [31] , [38] . As shown in Fig. 5a , the expression of mutp53 greatly increased the levels of RhoA-GTP but not the total RhoA in H1299 and p53 R172H/R172H MEF cells, and furthermore, knockdown of endogenous mutp53 greatly reduced the levels of RhoA-GTP but not the total RhoA in MDA-MB468 and SK-BR3 cells. We further investigated whether RhoA activation promotes GLUT1 translocation and the Warburg effect, and whether RhoA activation mediates mutp53’s GOF in stimulating the Warburg effect in cancer cells. Ectopic expression of RhoA by vectors in H1299 and p53−/− MEF cells greatly promoted the translocation of GLUT1 to the PM ( Fig. 5b ), and furthermore, greatly stimulated the Warburg effect ( Fig. 5c ). Consistently, RhoA knockdown by shRNA vectors or siRNA oligos clearly reduced the translocation of endogenous GLUT1 ( Fig. 5d ) and Myc-GLUT1 to the PM ( Fig. 5e–g ) and reduced the Warburg effect ( Fig. 5h–j ) in H1299, MDA-MB468 and p53 R172H/R172H MEF cells. Importantly, RhoA knockdown largely abolished the promoting effects of mutp53 on GLUT1 translocation to the PM ( Fig. 5d–g ) and the Warburg effect ( Fig. 5h–j ) in these cells. Similar results were observed in SK-BR3 cells ( Supplementary Fig. S3a–c ). Interestingly, consistent with the effect of mutp53 on GLUT2 and 3, RhoA did not show clear effect on the translocation of GLUT2 or 3 to the PM ( Supplementary Fig. S4 ). These results together clearly demonstrate a novel function of RhoA in tumorigenesis; RhoA activation promotes GLUT1 translocation to the PM, and therefore, promotes the Warburg effect in cancer cells, which is an important mechanism for mutp53 to stimulate the Warburg effect in cancer cells. 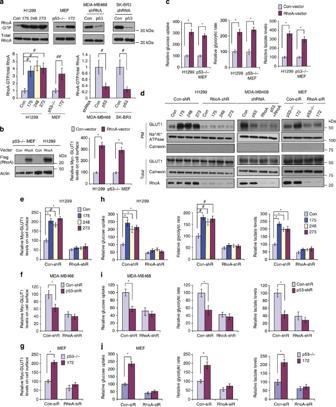Figure 5: Mutp53 stimulates the Warburg effect through activating RhoA. (a) Mutp53 enhanced RhoA activities represented by increased RhoA-GTP levels in cells. Upper panels: represented results of western blotting assays. Lower panels: relative RhoA-GTP/total RhoA levels in cells. Data are presented as mean±s.d. (n=4). (b) Ectopic expression of RhoA by expression vectors promoted the translocation of Myc-GLUT1 to the PM in H1299 andp53−/−MEF cells. (c) Ectopic expression of RhoA promoted the Warburg effect in H1299 andp53−/−MEF cells. (d) RhoA knockdown by shRNA or siRNA largely abolished the stimulating effects of mutp53 on the translocation of endogenous GLUT1 to the PM in H1299, MDA-MB468 and MEF cells. (e–g) RhoA knockdown largely abolished the stimulating effects of mutp53 on Myc-GLUT1 translocation to the PM in H1299 (e), MDA-MB468 (f) and MEF (g) cells. (h–j) RhoA knockdown largely abolished the stimulating effects of mutp53 on the Warburg effect in H1299 (h), MDA-MB468 (i) and MEF cells (j). Ind–j, two different shRNA vectors or siRNA oligos against RhoA were used and similar results were observed. Data are presented as mean±s.d. (n=4).##P<0.05;#P<0.01; *P<0.005; two-tailed Studentt-test. Figure 5: Mutp53 stimulates the Warburg effect through activating RhoA. ( a ) Mutp53 enhanced RhoA activities represented by increased RhoA-GTP levels in cells. Upper panels: represented results of western blotting assays. Lower panels: relative RhoA-GTP/total RhoA levels in cells. Data are presented as mean±s.d. ( n =4). ( b ) Ectopic expression of RhoA by expression vectors promoted the translocation of Myc-GLUT1 to the PM in H1299 and p53−/− MEF cells. ( c ) Ectopic expression of RhoA promoted the Warburg effect in H1299 and p53−/− MEF cells. ( d ) RhoA knockdown by shRNA or siRNA largely abolished the stimulating effects of mutp53 on the translocation of endogenous GLUT1 to the PM in H1299, MDA-MB468 and MEF cells. ( e – g ) RhoA knockdown largely abolished the stimulating effects of mutp53 on Myc-GLUT1 translocation to the PM in H1299 ( e ), MDA-MB468 ( f ) and MEF ( g ) cells. ( h – j ) RhoA knockdown largely abolished the stimulating effects of mutp53 on the Warburg effect in H1299 ( h ), MDA-MB468 ( i ) and MEF cells ( j ). In d – j , two different shRNA vectors or siRNA oligos against RhoA were used and similar results were observed. Data are presented as mean±s.d. ( n =4). ## P <0.05; # P <0.01; * P <0.005; two-tailed Student t -test. Full size image ROCK mediates the effect of mutp53 RhoA has been reported to regulate many proteins and different signalling pathways. Among them, ROCK is a direct downstream effector kinase of RhoA. ROCK has two isoforms, ROCK1 and ROCK2 (ROCK1/2) [30] , [38] . ROCK has been reported to regulate insulin-stimulated GLUT4 translocation and glucose uptake in fat and muscle tissues [39] , [40] , [41] . However, as the translocation regulation of GLUT1 and GLUT4 in cells is quite different and highly cell-type specific [25] , [32] , it is unclear whether ROCK activation can promote GLUT1 translocation and the Warburg effect in cancer cells. We investigated whether ROCK mediates mutp53 GOF in stimulating the Warburg effect. MYPT1 (myosin phosphatase target subunit 1) and MLC2 (myosin light chain 2) are two well-known downstream targets of ROCK, which can be phosphorylated by ROCK at Thr696 and Ser19, respectively [30] , [38] . First, we examined whether mutp53 enhances the activities of ROCK1/2 in cells by measuring the levels of phosphorylation at Thr696 of MYPT1 using enzyme immunoassays. Expression of mutp53 enhanced ROCK1/2 activities in H1299 and MEF cells, whereas knockdown of mutp53 reduced the ROCK1/2 activities in SK-BR3 and MDA-MB468 cells ( Fig. 6a ). This result was confirmed by western blotting assays showing that mutp53 expression clearly increased the phosphorylation of MYPT1 at Thr696 and MLC2 at Ser19 in H1299 cells ( Supplementary Fig. S5a ), whereas knockdown of endogenous mutp53 clearly reduced phosphorylation in MDA-MB468 cells ( Supplementary Fig. S5b ). This effect of mutp53 was largely abolished when RhoA or ROCK1/2 was knocked down by shRNA vectors or siRNA oligos ( Supplementary Fig. S5a–d ), indicating the mutp53 regulates the phosphorylation of MYPT1 and MLC2 through activation of the RhoA/ROCK signalling. 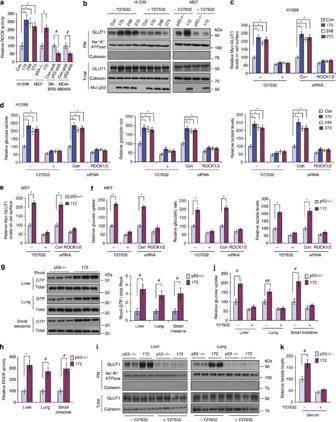Figure 6: Mutp53 stimulates the Warburg effect through ROCK activation bothin vitroandin vivo. (a) Mutp53 enhanced ROCK activities in H1299, MEF, SK-BR3 and MDA-MB468 cells as measured by enzyme immunoassays. (b) The ROCK inhibitor Y27632 (10 μM for 6 h) largely abolished the stimulating effect of mutp53 on GLUT1 translocation to the PM in H1299 and MEF cells. PM, plasma membrane; Total, whole-cell extracts. (c,d) Y27632 treatments and ROCK1/2 knockdown by siRNA largely abolished the stimulating effects of mutp53 on Myc-GLUT1 translocation to PM (c) and the Warburg effect (d) in H1299 cells. Cells transduced with pLPCX-Myc-GLUT1 vectors were transfected with siRNA oligos to simultaneously knock down ROCK1/2 at 24 h before assays. ROCK1/2 knockdown was confirmed by real-time PCR assays (Supplementary Fig. S5d). (e,f) Y27632 treatments (10 μM for 6 h) and ROCK1/2 knockdown largely abolished the stimulating effects of mutp53 on Myc-GLUT1 translocation (e) and the Warburg effect (f) inp53R172H/R172HMEF cells. (g) Enhanced RhoA-GTP levels in different tissues ofp53R172H/R172Hmice compared withp53−/−mice. Left panels: represented results of western blotting assays. Right panel: relative RhoA-GTP/total RhoA levels. Data are presented as mean±s.d. (n=6 mice with two time repeats). (h) Increased ROCK activities in different tissues ofp53R172H/R172Hmice compared withp53−/−mice. (i) Y27632 largely abolished the stimulating effect of R172H mutp53 on GLUT1 translocation to PM in different mouse tissues. Mice were killed at 3 h after Y27632 injection (i.p.; 10 μg g−1body weight) for assays. (j) Y27632 largely abolished the stimulating effect of R172H mutp53 on glucose uptake in different mouse tissues. Mice were injected (i.p.) with Y27632 at 3 h before glucose uptake assays. (k) Y27632 largely abolished the stimulating effect of R172H mutp53 on mouse serum lactate production. Inc–f, two different siRNA oligos against ROCK1 and ROCK2, respectively, were employed and similar results were observed. Ing–k, six mice per group were used for assays. Data are presented as mean±s.d. (n=4 ina–fandn=6 inh,j,k).##P<0.05;#P<0.01; *P<0.005; two-tailed Student’st-test. Figure 6: Mutp53 stimulates the Warburg effect through ROCK activation both in vitro and in vivo . ( a ) Mutp53 enhanced ROCK activities in H1299, MEF, SK-BR3 and MDA-MB468 cells as measured by enzyme immunoassays. ( b ) The ROCK inhibitor Y27632 (10 μM for 6 h) largely abolished the stimulating effect of mutp53 on GLUT1 translocation to the PM in H1299 and MEF cells. PM, plasma membrane; Total, whole-cell extracts. ( c , d ) Y27632 treatments and ROCK1/2 knockdown by siRNA largely abolished the stimulating effects of mutp53 on Myc-GLUT1 translocation to PM ( c ) and the Warburg effect ( d ) in H1299 cells. Cells transduced with pLPCX-Myc-GLUT1 vectors were transfected with siRNA oligos to simultaneously knock down ROCK1/2 at 24 h before assays. ROCK1/2 knockdown was confirmed by real-time PCR assays ( Supplementary Fig. S5d ). ( e , f ) Y27632 treatments (10 μM for 6 h) and ROCK1/2 knockdown largely abolished the stimulating effects of mutp53 on Myc-GLUT1 translocation ( e ) and the Warburg effect ( f ) in p53 R172H/R172H MEF cells. ( g ) Enhanced RhoA-GTP levels in different tissues of p53 R172H/R172H mice compared with p53−/− mice. Left panels: represented results of western blotting assays. Right panel: relative RhoA-GTP/total RhoA levels. Data are presented as mean±s.d. ( n =6 mice with two time repeats). ( h ) Increased ROCK activities in different tissues of p53 R172H/R172H mice compared with p53−/− mice. ( i ) Y27632 largely abolished the stimulating effect of R172H mutp53 on GLUT1 translocation to PM in different mouse tissues. Mice were killed at 3 h after Y27632 injection (i.p. ; 10 μg g −1 body weight) for assays. ( j ) Y27632 largely abolished the stimulating effect of R172H mutp53 on glucose uptake in different mouse tissues. Mice were injected (i.p.) with Y27632 at 3 h before glucose uptake assays. ( k ) Y27632 largely abolished the stimulating effect of R172H mutp53 on mouse serum lactate production. In c – f , two different siRNA oligos against ROCK1 and ROCK2, respectively, were employed and similar results were observed. In g – k , six mice per group were used for assays. Data are presented as mean±s.d. ( n =4 in a – f and n =6 in h , j , k ). ## P <0.05; # P <0.01; * P <0.005; two-tailed Student’s t -test. Full size image We further tested whether ROCK activation promotes GLUT1 translocation and the Warburg effect in cancer cells, and whether ROCK activation mediates mutp53’s role in stimulating GLUT1 translocation and the Warburg effect. Y27632, a widely used inhibitor for ROCK1/2 (refs 30 , 38 , 42 ), was employed to block ROCK1/2 activities in cells. Y27632 clearly reduced ROCK activities represented by the reduced phosphorylation of MYPT1 at Thr696 and MLC2 at Ser19 as measured by enzyme immunoassays and western blotting assays ( Supplementary Fig. S5e,f ). Furthermore, Y27632 largely abolished the promoting effect of mutp53 on ROCK activities in cells ( Supplementary Fig. S5e,f ). Notably, Y27632 greatly reduced the translocation of GLUT1 to the PM ( Fig. 6b,c ), and the Warburg effect in H1299 cells ( Fig. 6d ). Consistent results were observed in p53 R172H/R172H MEF cells ( Figs. 6b,e,f ). Importantly, Y27632 largely abolished the promoting effects of mutp53 on the translocation of GLUT1 to the PM ( Fig. 6b,c,e ), and the Warburg effect in these cells ( Fig. 6d,f ). Consistent results were observed in both SK-BR3 and MDA-MB468 cells ( Supplementary Fig. S6 ). To further confirm the role of ROCK in mediating the mutp53’s effect on GLUT1 translocation and the Warburg effect, the endogenous ROCK1/2 were knocked down by siRNA oligos. Consistent with the results of Y27632 treatments, knockdown of ROCK1/2 greatly reduced the GLUT1 translocation and the Warburg effect in cells, and furthermore, largely abolished the stimulating effects of mutp53 on GLUT1 translocation and the Warburg effect in H1299 ( Fig. 6c,d ), p53 R172H/R172H MEF ( Fig. 6e,f ) and MDA-MB468 cells ( Supplementary Fig. S6c,e ). These results clearly show that as a downstream effector of RhoA, ROCK mediates mutp53’s role in stimulating GLUT1 translocation and the Warburg effect in cancer cells. The phosphoinositide 3-kinase (PI3K)/AKT and ERK pathways, two pathways that are frequently activated in cancer, were reported to promote glucose uptake in cells [43] , [44] , [45] . To investigate whether these two pathways contribute to the promoting effects of mutp53 on the Warburg effect, we first examined whether mutp53 can activate these two pathways in these cell lines that we employed for this study by measuring the levels of phosphorylation of AKT at Thr473 and phosphorylation of ERK1/2 at Thr202/Tyr204, respectively. Mutp53 slightly increased the AKT activity in H1299 cells, which is consistent with a previous report [5] , but not in MDM-MB468 or MEF cells, suggesting that the activation of AKT by mutp53 is cell type and context dependent ( Supplementary Fig. S7a ) [46] . Mutp53 showed no clear effect on the ERK signalling in these cell lines ( Supplementary Fig. S7b ). To further test whether blocking the AKT and ERK signalling pathways affects the role of mutp53 in the Warburg effect, H1299 cells with or without mutp53 expression were treated with PI3K/AKT inhibitors, Wortmannin and LY294002 (refs 43 , 45 ), or ERK inhibitors, U0126 and PD98059 (ref. 44 ), and their impacts on mutp53’s effect on glucose uptake were examined. All these treatments greatly reduced the glucose uptake in H1299 cells. However, these treatments did not clearly affect the promoting effects of mutp53 on glucose uptake ( Supplementary Fig. S7c,d ). These results strongly suggested that the PI3K/AKT and ERK signalling pathways did not contribute significantly to the promoting effect of mutp53 on the Warburg effect in these cells. Insulin/IGF-1 (insulin-like growth factor-1) signalling has an important role in the regulation of the translocation of glucose transporters and glucose uptake in insulin-responsive muscle and fat tissues [25] . Activated IGF-1/IGF-1 receptor signalling also has an important role in cancer [47] . To investigate whether the activated insulin/IGF-1 signalling contributes to the effect of mutp53 on the GLUT1 translocation, H1299 cells were treated with insulin and IGF-1, respectively, to activate the insulin/IGF-1 signalling. Both insulin and IGF-1 moderately induced the GLUT1 protein expression (by ~2-fold at 8 h after treatments), and furthermore, slightly promoted GLUT1 translocation to the PM (by ~20–30% at 10 min, 4 and 8 h after treatments) in H1299 cells ( Supplementary Fig. S8 ). However, these effects were not mutp53-specific, as similar effects were observed in both H1299 cells with or without mutp53 expression. Furthermore, the effect of insulin and IGF-1 on GLUT1 translocation was much weaker compared with the effect of mutp53. These results suggested that activated insulin/IGF-1 signalling did not contribute significantly to the effect of mutp53 on GLUT1 translocation in H1299 cells. Mutp53 stimulates the Warburg effect via RhoA/ROCK in vivo We further investigated whether mutp53 stimulates the Warburg effect through the activation of the RhoA/ROCK signalling in vivo similar to what we observed in cultured cells. Indeed, the stimulating effect of mutp53 on the activities of RhoA and ROCK were also observed in p53 R172H/R172H mice. Compared with p53−/− mice, much higher levels of RhoA-GTP ( Fig. 6g ) and ROCK activities ( Fig. 6h and Supplementary Fig. S9 ) were observed in different tissues of p53 R172H/R172H mice, including the liver, lung and small intestine. Treating mice with Y27632 (intraperitoneal (i.p.) injection) clearly reduced the GLUT1 translocation to the PM ( Fig. 6i ) and glucose uptake ( Fig. 6j ) in different tissues and serum lactate levels ( Fig. 6k ). Importantly, Y27632 largely abolished mutp53’s effects on ROCK activation ( Supplementary Fig. S9 ), GLUT1 translocation ( Fig. 6i ), glucose uptake ( Fig. 6j ) and serum lactate levels ( Fig. 6k ). These results clearly show that the activated RhoA/ROCK signalling mediates the promoting effect of mutp53 on GLUT1 translocation and the Warburg effect in vivo . Mutp53 enhances actin polymerization Rho family proteins, including RhoA, induce actin polymerization and have an important role in vesicular trafficking, which is critical for the translocation of glucose transporters [29] , [48] , [49] . Actin polymerization, the assembly of actin monomers into filaments (polymeric actin or F-actin), has a critical role in vesicular trafficking [29] , [48] , [49] . ROCK has been reported to regulate insulin-stimulated GLUT4 translocation and glucose uptake in fat and muscle through the regulation of actin polymerization [39] . Interestingly, we found that mutp53 promoted actin polymerization. Expression of mutp53 clearly increased the levels of polymeric actin but not total actin in H1299 cells ( Fig. 7a ). This effect of mutp53 on actin polymerization can be largely abolished by inhibition of RhoA/ROCK signalling, including RhoA knockdown and Y27632 treatments ( Fig. 7a ). Cytochalasin D (Cyto D) and latrunculin B (Lat B), two widely used actin polymerization inhibitors [50] , [51] , which abolished the promoting effect of mutp53 on actin polymerization ( Fig. 7b ), also largely abolished the stimulating effects of mutp53 on the translocation of endogenous GLUT1 ( Fig. 7c ) and Myc-GLUT1 ( Fig. 7d ) to the PM in H1299 cells. Most importantly, Cyto D and Lat B largely abolished the stimulating effects of mutp53 on the Warburg effect in H1299 cells ( Fig. 7e ). These results were confirmed in p53 R172H/R172H MEF ( Fig. 7f–h ) and MDA-MB468 cells ( Fig. 7i–k ). These results strongly suggest that mutp53 can enhance actin polymerization through activating RhoA/ROCK signalling, which is one of the mechanisms that leads to the enhanced GLUT1 translocation to the PM and the Warburg effect in cancer cells. 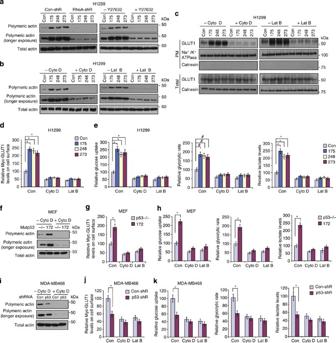Figure 7: Mutp53 promotes actin polymerization to promote GLUT1 translocation to the PM. (a) Mutp53 stimulated actin polymerization, which can be abolished by RhoA shRNA and ROCK inhibitor Y27632 (10 μM for 6 h) in H1299 cells expressing R175H, R248Q or R273H mutp53. (b) Actin polymerization inhibitors, cytochalasin D (Cyto D) and latrunculin B (LatB), abolished the promoting effect of mutp53 on actin polymerization in H1299 cells. (c,d) Cyto D and Lat B abolished the stimulating effect of mutp53 on the translocation of endogenous GLUT1 (c) and Myc-GLUT1 (d) to the PM in H1299 cells. Total, whole-cell extracts. (e) Cyto D and Lat B abolished the stimulating effect of mutp53 on the Warburg effect in H1299 cells. (f) Mutp53 promotes actin polymerization inp53R172H/R172HMEFs, which can be abolished by Cyto D. (g,h) Cyto D and Lat B abolished the stimulating effects of mutp53 on Myc-GLUT1 translocation to PM (g) and the Warburg effect (h) inp53R172H/R172HMEFs. (i) Knockdown of R273H mutp53 reduced actin polymerization in MDA-MB468 cells, which can be abolished by Cyto D. (j,k) Cyto D and Lat B abolished the stimulating effect of mutp53 on Myc-GLUT1 translocation to the PM (j) and the Warburg effect (k) in MDA-MB468 cells. Cells were treated with (+) or without (−) Cyto D (20 μM) or Lat B (10 μM) for 4 h before assays. Control groups (Con) were treated with dimethyl sulphoxide. Data are presented as mean±s.d. (n=3).#P<0.01; *P<0.005; two-tailed Student’st-test. Figure 7: Mutp53 promotes actin polymerization to promote GLUT1 translocation to the PM. ( a ) Mutp53 stimulated actin polymerization, which can be abolished by RhoA shRNA and ROCK inhibitor Y27632 (10 μM for 6 h) in H1299 cells expressing R175H, R248Q or R273H mutp53. ( b ) Actin polymerization inhibitors, cytochalasin D (Cyto D) and latrunculin B (LatB), abolished the promoting effect of mutp53 on actin polymerization in H1299 cells. ( c , d ) Cyto D and Lat B abolished the stimulating effect of mutp53 on the translocation of endogenous GLUT1 ( c ) and Myc-GLUT1 ( d ) to the PM in H1299 cells. Total, whole-cell extracts. ( e ) Cyto D and Lat B abolished the stimulating effect of mutp53 on the Warburg effect in H1299 cells. ( f ) Mutp53 promotes actin polymerization in p53 R172H/R172H MEFs, which can be abolished by Cyto D. ( g , h ) Cyto D and Lat B abolished the stimulating effects of mutp53 on Myc-GLUT1 translocation to PM ( g ) and the Warburg effect ( h ) in p53 R172H/R172H MEFs. ( i ) Knockdown of R273H mutp53 reduced actin polymerization in MDA-MB468 cells, which can be abolished by Cyto D. ( j , k ) Cyto D and Lat B abolished the stimulating effect of mutp53 on Myc-GLUT1 translocation to the PM ( j ) and the Warburg effect ( k ) in MDA-MB468 cells. Cells were treated with (+) or without (−) Cyto D (20 μM) or Lat B (10 μM) for 4 h before assays. Control groups (Con) were treated with dimethyl sulphoxide. Data are presented as mean±s.d. ( n =3). # P <0.01; * P <0.005; two-tailed Student’s t -test. Full size image Mutp53 GOF in the Warburg effect promotes tumorigenesis The Warburg effect has been recently demonstrated as a key contributor to tumour progression, and reversing the Warburg effect greatly compromised tumorigenicity of tumour cells [12] , [15] , [16] . We investigated whether stimulating the Warburg effect is an important mechanism contributing to mutp53’s role in tumorigenesis. Consistent with the reported GOF of mutp53 in tumorigenesis [4] , [5] , [6] , [7] , mutp53 promoted tumorigenesis in H1299 and MDA-MB468 cells. Expression of R175H, R248Q or R273H mutp53 in H1299 cells clearly promoted the anchorage-independent growth of the cells on soft agar ( Fig. 8a ), whereas knockdown of endogenous R273H mutp53 in MDA-MB468 cells clearly reduced the anchorage-independent growth of the cells ( Fig. 8b ). Furthermore, expression of mutp53 in H1299 cells clearly promoted the growth of xenograft tumours formed by H1299 cells in nude mice ( Fig. 8c–e ), whereas knockdown of endogenous R273H mutp53 in MDA-MB468 cells clearly reduced the growth of xenograft tumours formed by MDA-MB468 cells ( Fig. 8f ). Notably, knockdown of GLUT1 or RhoA by shRNA largely abolished the promoting effects of mutp53 on both anchorage-independent growth ( Fig. 8a,b ) and xenograft tumour growth ( Fig. 8c–f ) in H1299 and MDA-MB468 cells. 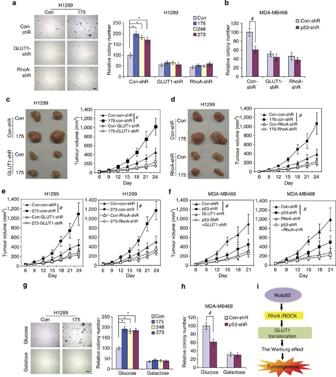Figure 8: Inhibition of glycolysis compromises mutp53 GOF in tumorigenesis. (a) Knockdown of GLUT1 or RhoA by shRNA vectors (GLUT1-shR or RhoA-shR) largely abolished the promoting effects of R175H, R248Q and R273H mutp53 on the anchorage-independent growth in H1299 cells. Left panel: represented images of colonies on soft agar in H1299 cells with R175H mutp53 expression and control cells. Scale bar, 100 μm. (b) Knockdown of GLUT1 or RhoA by shRNA vectors largely abolished the promoting effects of R273H mutp53 on the anchorage-independent growth in MDA-MB468 cells. (c,d) Knockdown of GLUT1 (c) or RhoA (d) by shRNA largely abolished the promoting effect of R175H mutp53 on the growth of xenograft tumours in H1299 cells. Left panels: represented images of tumours on day 24. Right panels: growth curves of xenograft tumours. (e) Knockdown of GLUT1 (left) or RhoA (right) by shRNA largely abolished the promoting effect of R273H mutp53 on the growth of xenograft tumours in H1299 cells. (f) Knockdown of GLUT1 (left) or RhoA (right) by shRNA largely abolished the promoting effect of R273H mutp53 on the growth of xenograft tumours in MDA-MB468 cells. (g,h) Culturing cells in media containing galactose but no glucose abolished the promoting effect of mutp53 on the anchorage-independent growth in H1299 (g) and MDA-MB468 (h) cells. Left panel ing: represented images of colonies on soft agar in H1299 cells with R175H mutp53 expression and control cells. Scale bar, 100 μm. (i) Model illustrating stimulation of the Warburg effect as a novel GOF of mutp53. Ina–h, two different shRNA vectors against each target gene, including GLUT1, RhoA and p53, were employed for all assays, and similar results were observed. Data are presented as mean±s.d. (n=10 forc–fandn=4 for the rest). *P<0.005;#P<0.01; two-tailed Student’st-test fora,b,g,h; analysis of variance followed by Student’st-tests forc–f. Figure 8: Inhibition of glycolysis compromises mutp53 GOF in tumorigenesis. ( a ) Knockdown of GLUT1 or RhoA by shRNA vectors (GLUT1-shR or RhoA-shR) largely abolished the promoting effects of R175H, R248Q and R273H mutp53 on the anchorage-independent growth in H1299 cells. Left panel: represented images of colonies on soft agar in H1299 cells with R175H mutp53 expression and control cells. Scale bar, 100 μm. ( b ) Knockdown of GLUT1 or RhoA by shRNA vectors largely abolished the promoting effects of R273H mutp53 on the anchorage-independent growth in MDA-MB468 cells. ( c , d ) Knockdown of GLUT1 ( c ) or RhoA ( d ) by shRNA largely abolished the promoting effect of R175H mutp53 on the growth of xenograft tumours in H1299 cells. Left panels: represented images of tumours on day 24. Right panels: growth curves of xenograft tumours. ( e ) Knockdown of GLUT1 (left) or RhoA (right) by shRNA largely abolished the promoting effect of R273H mutp53 on the growth of xenograft tumours in H1299 cells. ( f ) Knockdown of GLUT1 (left) or RhoA (right) by shRNA largely abolished the promoting effect of R273H mutp53 on the growth of xenograft tumours in MDA-MB468 cells. ( g , h ) Culturing cells in media containing galactose but no glucose abolished the promoting effect of mutp53 on the anchorage-independent growth in H1299 ( g ) and MDA-MB468 ( h ) cells. Left panel in g : represented images of colonies on soft agar in H1299 cells with R175H mutp53 expression and control cells. Scale bar, 100 μm. ( i ) Model illustrating stimulation of the Warburg effect as a novel GOF of mutp53. In a – h , two different shRNA vectors against each target gene, including GLUT1, RhoA and p53, were employed for all assays, and similar results were observed. Data are presented as mean±s.d. ( n =10 for c – f and n =4 for the rest). * P <0.005; # P <0.01; two-tailed Student’s t -test for a , b , g , h ; analysis of variance followed by Student’s t -tests for c – f . Full size image To further test this hypothesis, cells were cultured in media containing galactose instead of glucose to inhibit glycolysis [52] , [53] for anchorage-independent growth assays. Galactose enters glycolysis through the Leloir pathway, which occurs at a much lower rate than glucose entry into glycolysis. Consistent with previous reports [53] , galactose greatly reduced the anchorage-independent growth in H1299 ( Fig. 8g ) and MDA-MB468 cells ( Fig. 8h ). Notably, galactose largely abolished the promoting effect of mutp53 on the anchorage-independent growth in H1299 cells ( Fig. 8g ) and MDA-MB468 cells ( Fig. 8h ). Taken together, these results clearly show that inhibition of the Warburg effect or glycolysis greatly compromised mutp53 GOF in promoting tumorigenesis, and strongly suggest that mutp53 GOF in stimulating the Warburg effect promotes tumorigenesis. Recent studies have demonstrated that many tumour-associated mutp53 proteins gain new oncogenic functions to promote tumour cell proliferation, anti-apoptosis, metastasis and lipid metabolism [4] , [5] , [6] , [7] . However, the mechanism of mutp53 GOF in tumorigenesis is not well understood. Results from this study clearly demonstrate a novel GOF of mutp53 in both cultured cells and mutp53 knockin mice, that is, mutp53 stimulates the Warburg effect. This function of mutp53 is contrary to the function of wtp53 in repressing the Warburg effect, which was confirmed by our results in this study ( Figs 1 and 2 ). Mutp53 does not affect the expression of GLUT1, but promotes GLUT1 translocation to the PM. GLUT1 knockdown largely abolishes this stimulating effect of mutp53 on the Warburg effect in cells. Furthermore, mutp53 does not affect the expression or the PM translocation of GLUT2 or GLUT3. Knockdown of GLUT2 or GLUT3 clearly reduced the Warburg effect in cells, but did not clearly affect the stimulating effect of mutp53 on the Warburg effect. Currently, the mechanism by which mutp53 specifically regulates the translocation of GLUT1 in tumour cells remains unclear. These results strongly suggest that promoting the GLUT1 translocation to the PM is an important mechanism by which mutp53 stimulates the Warburg effect. GLUTs, including GLUT1–4, mediate the transport of glucose across the PM, a critical step for glucose metabolism. Each of these GLUTs displays distinct expression patterns in cells and tissues. For example, GLUT4 is specifically and highly expressed in fat and muscle tissues, and is responsive to insulin-stimulated glucose uptake in these two tissues. In contrast, GLUT1 is ubiquitously expressed and is responsible for the basal glucose uptake in various types of cells. The regulation of GLUTs translocation is different among GLUTs and the mechanisms appear to be highly cell type and context dependent [25] , [32] . For example, although translocation of GLUT4 is dramatically stimulated by insulin in fat and muscle cells, the translocation of GLUT1 is not markedly regulated by insulin [25] , [32] . It has been reported that the RhoA/ROCK signalling is involved in the regulation of the insulin-stimulated translocation of GLUT4 and glucose uptake [25] , [32] , [33] , [40] . However, it is unclear whether RhoA/ROCK signalling can regulate GLUT1 translocation and the basal glucose uptake in cells, especially in cells other than fat and muscle. Furthermore, it is unclear whether RhoA/ROCK activation in cancer cells promotes the Warburg effect in cancer cells. Results from this study clearly show that RhoA/ROCK can promote the translocation of GLUT1 to the PM and promote the basal glucose uptake in various cells. Furthermore, the activation of RhoA/ROCK signalling by mutp53 mediates mutp53’s role in promoting GLUT1 translocation and the Warburg effect in cancer cells. Inhibition of RhoA/ROCK signalling by knocking down RhoA or ROCK1/2, or by the ROCK inhibitor Y27632, all largely abolishes the stimulating effect of mutp53 on the GLUT1 translocation to the PM and the Warburg effect in cells. Thus, our results reveal that promoting the GLUT1 translocation to the PM to stimulate the Warburg effect in cancer cells is a novel mechanism by which the activated RhoA/ROCK signalling promotes tumorigenesis, especially in cells containing mutp53. The RhoA signalling is frequently activated in many types of cancer, which has a critical role in promoting tumour cell proliferation, invasion and metastasis [30] , [31] . In addition to our finding that mutp53 promotes the Warburg effect through RhoA activation, recent studies also showed that the activation of RhoA by mutp53 contributes to the GOF of mutp53 in tumour proliferation, invasion and metastasis [34] , [35] , [36] , [37] . These findings together indicate an important role of the RhoA signalling in mediating mutp53 GOF in cancer. However, it is still not well understood how mutp53 activates RhoA. As a small GTPase, RhoA activity is regulated by many positive and negative regulators, especially a group of Rho GEFs, Rho GAPs and Rho GDIs. Recently, it was reported that mutp53 activates RhoA through transcriptional upregulation of RhoGDI and Rho GEF-H1, two positive regulators for RhoA [34] , [35] , [36] . It will be of interest to examine whether mutp53 can regulate the expression of some other RhoA regulators to activate RhoA, including upregulation of additional positive regulators and/or downregulation of some negative regulators for RhoA. In addition to the transcription regulation, mutp53 can interact with other proteins to affect their functions, which contributes to the GOF of mutp53 in cancer [6] , [54] . It is possible that mutp53 interacts with some upstream regulators for RhoA to activate RhoA. Considering the important role of mutp53/RhoA signalling in tumorigenesis and potential therapeutic applications, future studies are needed to elucidate the molecular mechanism by which mutp53 activates RhoA. In summary, our results clearly demonstrate that stimulating the Warburg effect in tumour cells is a novel GOF of tumour-associated mutp53. Our results also reveal that mutp53 acts as an important mediator for the Warburg effect in cancer cells, which provides a new mechanism for the Warburg effect. Emerging evidence has strongly suggested that as a hallmark of tumour cells, metabolic changes in tumours, such as the Warburg effect, could be targeted for tumour therapy. Our results strongly suggest that targeting altered glucose metabolism could be a feasible therapeutic strategy for tumour carrying mutp53. Cells and vectors H1299, SK-BR3, MDA-MB468, H460, MCF7 and A549 cells were obtained from ATCC (Manassas, VA). The p53-null human lung H1299 cells were transduced with pLPCX-mutp53 retroviral vectors expressing R175H, R248Q and R273H mutp53, to establish cells with stable ectopic expression of mutp53. Human breast SK-BR3 cells expressing R175H mutp53 and MDA-MB468 cells expressing R273H mutp53 were transduced with shRNA vectors against p53 to establish cells with stable knockdown of endogenous mutp53 (ref. 21 ). pBABE-p53shRNA retroviral shRNA vectors against p53 was a generous gift from Dr R. Agami (The Netherlands Cancer Institute). The lentiviral shRNA vector against p53 (TRCN0000003756) were purchased from Sigma. Control cells were transduced with empty vectors. p53−/− and p53 R172H/R172H MEF cells were established following the published method [55] . RhoA expression vector pLPCX-Flag-RhoA was constructed by using Flag-RhoA DNA fragment from pCMV5-Flag-RhoA (Addgene). Lentiviral shRNA vectors against human GLUT1 (V3LHS_321625 and V3LHS_321626), human GLUT3 (V3LHS_323130 and V3LHS_323134) and human RhoA (V3LHS_646048 and V3LHS_642222) were purchased from Open Biosystems (Huntsville, AL). siRNA oligos against ROCK1 (for human: HSC.RNAI.N005406.12.1 and HSC.RNAI.N005406.12.2; for mouse: MMC.RNAI.N009071.12.1 and MMC.RNAI.N009071.12.3), ROCK2 (for human: HSC.RNAI.N004850.12.1 and HSC.RNAI.N004850.12.2; for mouse: MMC.RNAI.N009072.12.1 and MMC.RNAI.N009072.12.4), mouse GLUT1 (MMC.RNAI.N011400.12.4 and MMC.RNAI.N011400.12.5) and mouse GLUT3 (MMC.RNAI.N011401.12.2 and MMC.RNAI.N011401.12.4) were purchased form Integrated DNA Technologies. siRNA oligos against mouse GLUT2 (5′-AAGUUGGAAGAGGAAGUCATT-3′ and 5′-CGGAAAGCUGCCAUUAACUTT-3′) were synthesized by Sigma. To avoid off-target effects, two different shRNA vectors or siRNA oligos against each gene were employed. For treatment of ROCK inhibitor Y27632, cells were treated with Y27632 (5, 10 and 20 μM; stock solution was prepared in H 2 O) for 6 h before assays. For treatments of AKT inhibitors, cells were treated with Wortmannin (0.5, 1 and 2 μM) or LY294002 (10, 20 and 30 μM) for 3 h before assays. For treatments of ERK inhibitors, cells were treated with U0126 (0.5, 1 and 2 μM) or PD98059 (5, 10 and 20 μM) for 2 h before assays. For treatments of IGF-1 and insulin, cells were serum starved for 12 h before they were treated with IGF-1 (50 and 100 ng ml −1 ) or insulin (50 and 100 nM) for 10 min, 4 h and 8 h before assays. In vivo glucose uptake assays and serum lactate measurements Assays for glucose uptake in mouse tissues were performed as described [56] , [57] . Briefly, 5-week-old male p53+/+ , p53−/− and p53 R172H/R172H C57BL6/J mice [8] (generous gifts from Dr Gigi Lozano) were injected (i.p.) with 3 H-2-deoxyglucose (1 μCi per g body weight) and tissues were collected at 1.5 h after injection to measure the levels of 3 H-2-deoxyglucose-6-phosphate accumulated in tissues. To study the effect of ROCK inhibitor Y27632 on glucose uptake of tissues, mice were injected (i.p.) with Y27632 (10 μg per g body weight) or PBS at 3 h before injection (i.p.) of 3 H-2-deoxyglucose. The lactate levels in serum were determined by using a lactate Assay Kit according to the manufacturer’s instruction (Biovision). All mouse experiments were approved by the Institutional Animal Care and Use Committee of Rutgers University. Measurements of glucose uptake in cells Glucose uptake was measured by measuring the uptake of 3 H-2-deoxyglucose by cells [21] , [58] . Briefly, cells cultured in 12-well plates were pre-incubated in glucose-free media for 30 min. 3 H-2-deoxyglucose (1 μCi per well) was then added to the cells and incubated for 30 min before cells were washed with PBS and lysed in 1% SDS. The radioactivity of cell lysates was determined in a liquid scintillation counter and normalized to the protein concentrations of cell lysates. Measurements of glycolytic rates in cells The glycolytic rate was measured by monitoring the conversion of 5- 3 H-glucose to 3 H-H 2 O (refs 19 , 21 ). Briefly, cells (1 × 10 6 ) were washed in PBS and then resuspended in 1 ml of Krebs buffer without glucose for 30 min at 37 °C. Cells were then resuspended in 0.5 ml of Krebs buffer containing 10 mM glucose and 5 μCi of 5-[ 3 H]glucose for 1 h. Triplicate 100 μl aliquots were transferred to uncapped PCR tubes containing 100 μl of 0.2 N HCl, and a tube was transferred to a scintillation vial containing 0.5 ml of H 2 O. The scintillation vials were sealed and left for 48 h to allow diffusion to occur. The amounts of diffused and undiffused 3 H were determined in a liquid scintillation counter. Measurements of lactate production in cells Cells were cultured in fresh phenol red-free media and incubated for 12–24 h before the culture media were collected. The lactate levels were determined by using lactate Assay Kits according to the manufacturer’s instruction (Biovision) and normalized with cell number [21] . Western blotting assays Standard western blotting assays and following antibodies were used to analyse protein expression: GLUT1 (Abcam; 1:4,000), GLUT2 (Abcam; 1:2,000), GLUT3(Abcam; 1:2,000), GLUT4 (Santa Cruz; 1:2,000), RhoA (Millipore; 1:2,000), p53 (Santa Cruz; 1:1,000), β-actin (Sigma; 1:20,000), Na + /K + ATPase (Novus; 1:3,000), Calnexin (Abcam; 1:5,000), Flag (Sigma; 1:10,000), Myc (Roche; 1:1,000), p-AKT (Ser473; Cell Signaling; 1:1,000), AKT (Santa Cruz; 1:4,000), p-ERK1/2 (Cell Signaling; 1:2,000), ERK1/2 (Cell Signaling; 1:2,000), p-MYPT1 (Thr696; EMD Millipore; 1:2,000), MYPT1 (Cell Signaling; 1:2,000), p-MLC2 (Ser19; Cell Signaling; 1:1,000) and MLC2 (Cell Signaling; 1:2,000). The full blots are shown in supplementary Fig. S10 . Quantitative real-time PCR assays Total RNA was prepared with the RNeasy Kit (Qiagen). Complementary DNA was prepared using a TaqMan reverse-transcription kit, and real-time PCR was performed with TaqMan PCR mixture (Applied Biosystems, Foster City, CA) according to standard protocols [21] . The Taqman primers for human ROCK1 (Hs01127699_m1), human ROCK2 (Hs00178154_m1), human actin (Hs99999903_m1), mouse ROCK1 (Mm00485745_m1), mouse ROCK2 (Mm01270843_m1) and mouse actin (Mm01205647_g1) were purchased from Applied Biosystems. The expression of ROCK1 and ROCK2 in cells was normalized to the expression of actin gene. Assays for RhoA and ROCK activities For RhoA activity analysis, glutathione- S -transferase–Rhotekin Rho-binding domain pull-down assays were performed with Rho activity kits (Millipore) to measure the levels of GTP-bound RhoA (RhoA-GTP) in cells [59] . The Rhotekin Rho-binding domain of the Rho effector protein Rhotekin binds specifically to the RhoA-GTP. The levels of precipitated RhoA-GTP were measured by western blotting assays using a RhoA antibody, and normalized to total RhoA levels in cells. The ROCK activity was measured by enzyme immunoassays using ROCK activity assay kits (Millipore). In brief, ROCK1/2 were immunoprecipitated from cell lysates and added to 96-well plates precoated with recombinant MYPT1, which contains a Thr696 residue that can be phosphorylated by ROCK1/2 (ref. 59 ). The levels of MYPT1 phosphorylation on Thr696, which represent the ROCK1/2 activities, were detected with a phospho-MYPT1-Thr696 antibody (1:1,000) and an horseradish-peroxidase-conjugated secondary detection antibody (1:2,000). Analysis of endogenous levels of GLUTs on the PM The PM fraction of cells was isolated according to standard protocols [60] , [61] . Briefly, the PM fraction was separated from the other membrane fraction of cells, which includes the endoplasmic reticulum (ER). The expression levels of GLUT1, 2 and 3 in the PM fraction were measured by western blotting assays. A PM protein Na + /K + ATPase was detected as an internal standard. Calnexin, an ER membrane protein, was detected to exclude the contamination of PM by the other membrane fractions, which includes the ER. The whole-cell extracts were used to measure the total GLUT1, 2 and 3 in cells. Analysis of the levels of Myc-tagged GLUTs on the PM The pEGP-Myc-GLUT1 and pcDNA3-Myc-GLUT2 vectors, which express GLUT1 and GLUT2 with Myc tag in their first exofacial loops, respectively, (generous gifts from Dr Jeffrey Pessin), were used to construct pLPCX-Myc-GLUT1 and pLPCX-Myc-GLUT2 vectors, respectively. The pLPCX-Myc-GLUT3 vector expressing GLUT3 with Myc tag in its first exofacial loop was constructed by PCR amplification. The levels of Myc-GLUT1, 2 and 3 on the cell surface and in whole cells were measured by IF staining in a flow cytometry [62] , [63] . Briefly, at 48 h after cells were transduced with pLPCX-Myc-GLUT1, 2 or 3 vectors, cells were blocked in PBS with 2% fetal bovine serum and stained with a Myc antibody (Roche) to detect Myc-GLUT1, 2 or 3 on cell surface in a flow cytometry. To determine the total levels of Myc-GLUT1, 2 or 3 in cells, cells were fixed with 2% paraformaldehyde and permeabilized with 0.2% Triton X-100 before staining. The relative levels of Myc-GLUT 1, 2 or 3 on cell surface were calculated after normalization with their total levels in cells. Cells transduced with empty pLPCX vectors were employed as negative controls. Immunofluorescence staining IF staining of cells were performed according to standard protocols [21] , [22] . In brief, cells cultured on coverslips were washed with ice-cold PBS and fixed with methanol. Cells were permeabilized with PBS containing 0.2% Triton X-100. The cells expressing Myc-GLUT1 were incubated with anti-myc antibodies (9E10, Roche; 1:100) for overnight followed by Alexa Fluor 488-conjugated goat secondary antibody (Invitrogen; 1:200) for 1 h. The coverslips were mounted in Vectashield (Vector Laboratories) and examined by a confocal laser-scanning microscopy. Actin polymerization assays The polymeric actin fraction was isolated from cells according to standard protocols [64] . Briefly, cells were homogenized in 400 μl of lysis and F-actin stabilization buffer (50 mM PIPES at pH 6.9, 50 mM NaCl, 5 mM MgCl 2 , 5 mM EGTA, 5% glycerol, 0.1% NP-40, 0.1% Triton X-100, 0.1% Tween-20, 0.1% β-mercaptoethanol, 1 mM ATP and protease inhibitor cocktail) for 30 min at 37 °C. Following centrifugation (300 g, 5 min), half of the supernatant was transferred and centrifuged at 100,000 g (60 min, 37 °C) to pellet polymeric actin. The pellet containing polymeric actin was resuspended in 200 μl of ice-cold water containing 10 μM Cyto D. The polymeric actin samples were then diluted in 4 × SDS sample buffer for western blotting assays. A monoclonal anti-actin antibody (Sigma) was used to detect polymeric actin. The whole-cell extracts from the same amount of cells used for polymeric actin fraction isolation were used for the western blotting assays to measure the levels of total actin in cells. For treatments of actin polymerization inhibitors, cells were treated with Cyto D (5–20 μM) or Lat B (1–10 μM) for 4 h before assays. Control groups were treated with dimethyl sulphoxide. Anchorage-independent growth assays Anchorage-independent growth assays were performed in dishes coated with media containing 0.6% agarose. Cells were seeded on top of this layer in media containing 0.3% agarose. Colonies were stained and counted after 2–3 weeks. For galactose treatment, cells were cultured in media containing galactose (25 mM) but no glucose. Xenograft tumorigenicity assays Seven-week-old BALB/c nu/nu male athymic nude mice (Taconic) were used for xenograft tumorigenicity assays [65] . Cells (5 × 10 6 −1 × 10 7 in 0.2 ml PBS) were injected (subcutaneously) into nude mice ( n =10 per group). After injection, mice were examined and tumour volumes were measured three times per week for 3–4 weeks. Tumour volume=1/2 (length × width 2 ). Statistical analysis The differences in tumour growth among groups were analysed for statistical significance by analysis of variance, followed by Student’s t -tests using GraphPad Prism software. All other P -values were obtained using two-tailed Student t -tests; * P <0.005; # P <0.01; ## P <0.05. How to cite this article: Zhang, C. et al . Tumour-associated mutant p53 drives the Warburg effect. Nat. Commun. 4:2935 doi: 10.1038/ncomms3935 (2013).